Transcription factors FOXG1 and Groucho/TLE promote glioblastoma growth Glioblastoma (GBM) is the most common and deadly malignant brain cancer, with a median survival of <2 years. GBM displays a cellular complexity that includes brain tumour-initiating cells (BTICs), which are considered as potential key targets for GBM therapies. Here we show that the transcription factors FOXG1 and Groucho/TLE are expressed in poorly differentiated astroglial cells in human GBM specimens and in primary cultures of GBM-derived BTICs, where they form a complex. FOXG1 knockdown in BTICs causes downregulation of neural stem/progenitor and proliferation markers, increased replicative senescence, upregulation of astroglial differentiation genes and decreased BTIC-initiated tumour growth after intracranial transplantation into host mice. These effects are phenocopied by Groucho/TLE knockdown or dominant inhibition of the FOXG1:Groucho/TLE complex. These results provide evidence that transcriptional programmes regulated by FOXG1 and Groucho/TLE are important for BTIC-initiated brain tumour growth, implicating FOXG1 and Groucho/TLE in GBM tumourigenesis. Glioblastoma (GBM; World Health Organization grade IV glioma) is the most malignant and frequent primary brain cancer, representing up to 60% of all astrocyte-lineage tumours [1] , [2] , [3] . GBM patients have a median survival time of ~15 months, because the aggressive and recurring nature of this cancer can only be temporarily contained by surgical resection followed by combined radiotherapy and chemotherapy [1] , [2] , [3] . GBM is a highly heterogeneous cancer containing a combination of cells exhibiting varying degrees of differentiation [4] , [5] . It is hypothesized that among the most poorly differentiated GBM cells are cells endowed with stem-like properties, namely the ability to maintain extended self-renewal and give rise to rapidly proliferating progenies, potential for multilineage differentiation and capacity to propagate cancers resembling the parental tumour [4] , [5] , [6] , [7] , [8] , [9] . GBM cells with these characteristics are postulated to act as tumour-forming cells and are commonly referred to as brain tumour-initiating cells (BTICs) [4] , [5] , [6] , [7] , [8] , [9] , [10] . BTICs are also regarded as a possible culprit for GBM recurrence because of their suggested ability to repopulate cancer after surgical removal of the primary tumour. Because of these predicted properties, BTICs are hypothesized to represent the chemotherapy-resistant cell population within GBM, as their postulated slow proliferation rate, combined with a more effective drug-resistance capacity, is thought to make them refractory to antimitotic drugs [4] , [5] , [10] . BTICs thus represent a therapeutically attractive target for GBM treatment strategies. BTICs are thought to share several properties with normal neural stem/progenitor cells (NSPCs), including prolonged self-renewal ability, pluripotency and tissue repopulating potential. However, they differ from the latter in a number of ways, including the presence of genetic abnormalities and aberrant gene expression patterns, the ability to proliferate independent of mitogens, impaired differentiation potential, and tumour-forming capacity [11] , [12] , [13] . These observations suggest that the tumourigenic potential of BTICs may result, at least in part, from the perturbation of molecular mechanisms that normally regulate the balance between proliferation and differentiation in NSPCs. In potential agreement with this possibility, a number of cell intrinsic factors that maintain the NSPC state under normal conditions, including sex-determining region Y-box2 (SOX2), B lymphoma Mo-MLV insertion region 1 homologue (BMI1) and oligodendrocyte transcription factor 2 (OLIG2), are expressed in GBM and have been implicated in the maintenance and tumourigenicity of BTICs [9] , [14] , [15] , [16] , [17] . It is therefore anticipated that our understanding of the processes that contribute to cellular transformation in GBM will be facilitated by improved knowledge of the molecular pathways that promote BTIC propagation and inhibit their differentiation potential. The mouse gene Foxg1 , which encodes a DNA-binding transcription factor belonging to the forkhead protein family, is a key regulator of NSPC biology in both the developing and adult forebrain. Foxg1 acts to maintain the NSPC state at the expense of neural cell differentiation and its inactivation causes a dramatic perturbation of cerebral cortex development as a result of premature NSPC differentiation [18] , [19] , [20] . Conversely, Foxg1 overexpression in cultured NSPCs results in a lasting expansion of the undifferentiated cell pool, with a concomitant blockade of neural differentiation [21] , [22] . The FoxG1 protein acts, at least in part, by forming transcription repression complexes with corepressors of the Groucho/transducin-like Enhancer of split (TLE) family (hereafter, the four members of this family will be referred to as TLE1-4) [23] , [24] , [25] . TLE proteins are global transcriptional corepressors that participate in mechanisms that maintain the stem/progenitor cell state and inhibit differentiation in a variety of tissues [26] , [27] . It was reported that the human orthologue of FoxG1, termed FOXG1, is expressed in GBM [28] , [29] , but its involvement in GBM tumourigenesis was not investigated. In this study, we sought to characterize the expression and function of FOXG1 and its transcriptional partner, TLE, in GBM and BTICs. Our results provide evidence that elevated FOXG1 and TLE1 expression is a common event in human GBM and is associated with worse overall patient survival. FOXG1 and TLE1 are coexpressed, and form a complex, in BTICs where their activity is important for sustained proliferation. More importantly, inhibition of FOXG1 and TLE functions decreases BTIC-initiated brain tumour growth. Together, these findings implicate transcriptional programmes regulated by FOXG1 and TLE proteins in GBM tumourigenesis. Elevated FOXG1 expression correlates with poor GBM prognosis Analysis of the GeneSapiens database, which contains information on messenger RNA expression levels for >11,000 genes in >10,000 different human tissue samples [30] , showed that FOXG1 mRNA was preferentially expressed in the nervous tissue in healthy cases, in agreement with the specific forebrain expression of Foxg1 in the mouse nervous system [18] . In cancer samples, FOXG1 expression was elevated in glioma compared with other tumours ( Fig. 1a ). Immunohistochemistry on human GBM tissues ( n =30 stained specimens) using a validated anti-FOXG1 antibody ( Supplementary Fig. S1 ) showed that approximately half of all cells in GBM specimens expressed FOXG1, a fraction that was considerably higher than in normal adult brain ( Fig. 1b,c ). Grade II and III glioma displayed progressively higher numbers of FOXG1-positive cells compared with control adult brain, but these numbers were lower than in GBM. Western blot analysis confirmed that the FOXG1 protein was expressed at significantly higher levels in GBM compared with that in normal brain ( Fig. 1d ). On the basis of these observations, we assessed the significance of FOXG1 expression with regard to the GBM patient population by examining the REMBRANDT (Repository of Molecular Brain Neoplasia Data) database of the National Cancer Institute [31] . Comparison of overall survival of GBM patients ( n =181) with different levels of FOXG1 expression revealed a significant decrease in overall survival in the presence of elevated FOXG1 expression and a better survival with lower FOXG1 levels ( Fig. 1e ). Taken together, these results provide evidence that an increased number of FOXG1-expressing cells is a common event in GBM and that elevated FOXG1 levels are correlated with a poor prognosis. 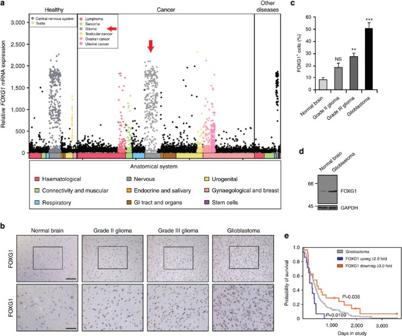Figure 1: Elevated FOXG1 expression in GBM correlates with poor prognosis. (a) Body-wide expression ofFOXG1across the GeneSapiens database, with each dot representing expression in a single sample. Anatomical sources of examined samples are indicated with coloured bars below the gene plot, with corresponding legends also shown. Anatomical samples with higher-than-averageFOXG1expression or an outlier expression profile are shown coloured. Vertical red arrow points toFOXG1expression in glioma. (b) Formalin-fixed, paraffin-embedded sections from normal brain or glioma of increasing grade were subjected to immunohistochemistry with a validated anti-FOXG1 antibody, followed by counterstaining with haematoxylin. Boxed areas in the top row define regions shown at higher magnification in the bottom row. A representative image is shown for each group. Scale bars, 100 μm (top row) and 50 μm (bottom row). (c) Quantification of the number of FOXG1-positive nuclei in normal brain or glioma specimens. Data are represented as mean±s.e.m. (grade II glioma, NS, not significant,n=12; grade III glioma,P=1.2 × 10−3,n=16; GBM,P<1.0 × 10−4,n=16; normal brain,n=13; analysis of variance (ANOVA)). (d) Western blot analysis of FOXG1 expression in normal brain and GBM tissue extracts. Expression of GAPDH is shown as loading control. Molecular size markers are indicated in kDa. One representative western blotting result is shown (n≥3). (e) Kaplan–Meier curves comparing survival among GBM patients. Survival curves are shown for patients with tumours exhibiting either high (blue curve) or low (orange curve)FOXG1mRNA levels compared with all GBM patients (grey curve). Data were obtained from the Rembrandt Database of the National Cancer Institute. Statistical analysis (P-value calculated using Mantel–Cox test) for high versus all, or low versus all,FOXG1levels is shown next to the corresponding curves. Figure 1: Elevated FOXG1 expression in GBM correlates with poor prognosis. ( a ) Body-wide expression of FOXG1 across the GeneSapiens database, with each dot representing expression in a single sample. Anatomical sources of examined samples are indicated with coloured bars below the gene plot, with corresponding legends also shown. Anatomical samples with higher-than-average FOXG1 expression or an outlier expression profile are shown coloured. Vertical red arrow points to FOXG1 expression in glioma. ( b ) Formalin-fixed, paraffin-embedded sections from normal brain or glioma of increasing grade were subjected to immunohistochemistry with a validated anti-FOXG1 antibody, followed by counterstaining with haematoxylin. Boxed areas in the top row define regions shown at higher magnification in the bottom row. A representative image is shown for each group. Scale bars, 100 μm (top row) and 50 μm (bottom row). ( c ) Quantification of the number of FOXG1-positive nuclei in normal brain or glioma specimens. Data are represented as mean±s.e.m. (grade II glioma, NS, not significant, n =12; grade III glioma, P =1.2 × 10 −3 , n =16; GBM, P <1.0 × 10 −4 , n =16; normal brain, n =13; analysis of variance (ANOVA)). ( d ) Western blot analysis of FOXG1 expression in normal brain and GBM tissue extracts. Expression of GAPDH is shown as loading control. Molecular size markers are indicated in kDa. One representative western blotting result is shown ( n ≥3). ( e ) Kaplan–Meier curves comparing survival among GBM patients. Survival curves are shown for patients with tumours exhibiting either high (blue curve) or low (orange curve) FOXG1 mRNA levels compared with all GBM patients (grey curve). Data were obtained from the Rembrandt Database of the National Cancer Institute. Statistical analysis ( P -value calculated using Mantel–Cox test) for high versus all, or low versus all, FOXG1 levels is shown next to the corresponding curves. Full size image FOXG1 is expressed in poorly differentiated GBM cells Double-label immunofluorescence analysis of paraffin-embedded human GBM specimens revealed that 12.64±2.72% of FOXG1-expressing cells in GBM coexpressed the proliferating cell marker Ki67 (mean±s.e.m. ; n =5; Fig. 2a ). Conversely, 66.34±6.25% of all Ki67-positive cells in GBM coexpressed FOXG1 (mean±s.e.m. ; n =5). This finding showed that FOXG1 expression was not merely correlated with actively proliferating cells and suggested that at least some of the FOXG1-positive cells might have features of less-proliferative NSPC-like cells. Consistent with this possibility, numerous FOXG1-positive cells in GBM specimens coexpressed proteins present in NSPCs, including BMI1, SOX2, OLIG2 and NESTIN [9] , [10] , [11] , [12] , [13] , [14] , [15] , [16] ( Fig. 2a ). Specifically, we observed that 58.52±6.22% of FOXG1-positive cells in GBM coexpressed OLIG2 (mean±s.e.m. ; n =5). Moreover, 62.95±7.03% of FOXG1-positive cells also expressed CD44 in the GBM cases examined ( Fig. 2a ). CD44 was shown to be expressed at high frequency in GBM of the mesenchymal subtype and was proposed as a marker of cancer stem-like cells in breast cancer [32] , [33] , [34] . We also detected overlapping expression of FOXG1 and glial fibrillary acidic protein (GFAP) in GBM ( Fig. 2b ). In normal brain, GFAP is expressed in many parenchymal astrocytes, in addition to cells with NSPC-like features located in specific stem cell niches. However, we could not detect cells with overlapping FOXG1 and GFAP expression in normal brain parenchyma ( Fig. 2b ). In contrast, all FOXG1-positive cells in control brain, as well as non-cancerous inflammatory brain conditions, coexpressed the neuronal marker protein NeuN [20] ( Supplementary Fig. S2 ). Taken together, these findings show that FOXG1 is frequently expressed in poorly differentiated astroglial cells in GBM, in contrast to its expression in neuronal cells in non-cancerous brain tissues. 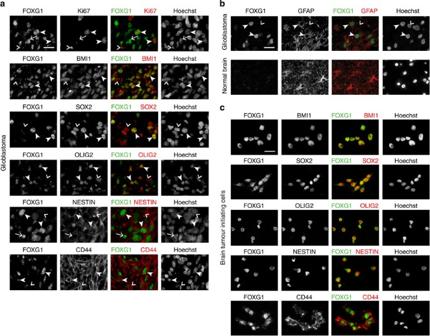Figure 2: FOXG1 is expressed in a hierarchy of poorly differentiated GBM cells. (a) Double-labelling immunofluorescence analysis of the expression of FOXG1 and either Ki67, BMI1, SOX2, OLIG2, NESTIN or CD44 using formalin-fixed, paraffin-embedded (FFPE) sections from GBM surgical specimens. Nuclei were counterstained with Hoechst. Closed arrowheads point to examples of cells with overlapping expression of FOXG1 and indicated marker protein. Arrows point to examples of cells positive for FOXG1 but not for the marker under study. Open arrowheads point to examples of cells negative for FOXG1 but positive for the indicated marker protein. Scale bars, 20 μm. (b) Double-labelling immunofluorescence analysis of the expression of FOXG1 and GFAP using FFPE sections from either GBM or control adult brain. Nuclei were counterstained with Hoechst. Scale bar, 20 μm. (c) Double-labelling immunofluorescence analysis of the expression of FOXG1 and either BMI1, SOX2, OLIG2, NESTIN or CD44 in cultured BTIC line BT012. Nuclei were counterstained with Hoechst. Scale bar, 20 μm. In all depicted studies, a representative set of images is shown (n≥3). Figure 2: FOXG1 is expressed in a hierarchy of poorly differentiated GBM cells. ( a ) Double-labelling immunofluorescence analysis of the expression of FOXG1 and either Ki67, BMI1, SOX2, OLIG2, NESTIN or CD44 using formalin-fixed, paraffin-embedded (FFPE) sections from GBM surgical specimens. Nuclei were counterstained with Hoechst. Closed arrowheads point to examples of cells with overlapping expression of FOXG1 and indicated marker protein. Arrows point to examples of cells positive for FOXG1 but not for the marker under study. Open arrowheads point to examples of cells negative for FOXG1 but positive for the indicated marker protein. Scale bars, 20 μm. ( b ) Double-labelling immunofluorescence analysis of the expression of FOXG1 and GFAP using FFPE sections from either GBM or control adult brain. Nuclei were counterstained with Hoechst. Scale bar, 20 μm. ( c ) Double-labelling immunofluorescence analysis of the expression of FOXG1 and either BMI1, SOX2, OLIG2, NESTIN or CD44 in cultured BTIC line BT012. Nuclei were counterstained with Hoechst. Scale bar, 20 μm. In all depicted studies, a representative set of images is shown ( n ≥3). Full size image On the basis of these results, and the previous demonstration that mouse FoxG1 is expressed in NSPCs in the developing and adult brain [18] , [19] , [20] , [21] , we next assessed whether FOXG1 was expressed in primary cultures of GBM-derived BTICs [9] , [12] , [13] . Specifically, we examined FOXG1 expression in five previously characterized human patient-derived primary BTIC lines that were rigorously selected based on their tumour-propagation ability in vivo , as well as capacity for continued propagation under low cell-density conditions and multilineage potential in vitro [12] . FOXG1 was expressed in all of these BTIC lines ( Supplementary Fig. S3a ). More importantly, FOXG1 was coexpressed with BMI1, SOX2, OLIG2, NESTIN and CD44 in these cells ( Fig. 2c and Supplementary Fig. S3b ). Together, these results provide evidence that FOXG1 is expressed in a hierarchy of poorly differentiated GBM cells expressing NSPC markers in vivo and in primary cultures of BTICs in vitro . FOXG1 silencing impairs proliferation in cultured BTICs Mouse FoxG1 plays a key role in the maintenance of embryonic and postnatal NSPCs [18] , [19] , [20] , [21] . We therefore investigated whether human FOXG1 might be important for the propagation of GBM-derived BTICs in vitro . At first, neurosphere formation assays were performed to monitor the ability of cultured BTICs to give rise to clones (neurospheres) of undifferentiated progeny cells under low cell-density (10–100 cells per ml) clonogenic conditions [12] , [35] . We compared neurosphere formation frequency after lentiviral-mediated delivery of either non-silencing (that is, ‘scrambled’) short hairpin RNA (shRNA) or FOXG1 shRNA reagents. Two separate FOXG1 shRNA reagents were used to control for nonspecific off-site effects (these reagents will be hereafter termed FOXG1 shRNA 1 and 2). Expression of either of these FOXG1 shRNAs resulted in a marked knockdown of FOXG1 protein expression in three separate BTIC lines, referred to as BT012, BT025 and BT048 (ref. 12 ; Fig. 3a and Supplementary Fig. S4a ). This effect was correlated with a significant decrease in neurosphere formation frequency compared with cells transduced with non-silencing shRNA, indicative of decreased BTIC propagation ability as a result of FOXG1 knockdown ( Fig. 3b and Supplementary Fig. S4b ). 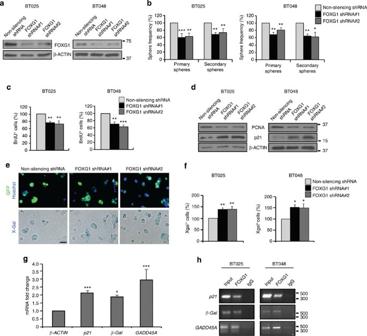Figure 3: FOXG1 silencing impairs proliferation in cultured BTICs. (a) Western blot analysis of FOXG1 in BTIC lines BT025 and BT048 after transduction with lentivirus expressing non-silencing shRNA orFOXG1shRNA 1 and 2 reagents. β-ACTIN is shown as loading control. Molecular size markers are indicated in kDa. One representative western blot result is shown in each case (n≥3). (b) Quantification of the sphere-forming ability of non-silenced or FOXG1-silenced BT025 and BT048 cells passaged for two generations (mean±s.e.m.; BT025: shRNA 1, primary spheres,P=2.0 × 10−4,n=10, secondary spheres,P=2.3 × 10−3,n=6; shRNA 2, primary spheres,P=9.1 × 10−3,n=3, secondary spheres,P=5.5 × 10−3,n=3; BT048: shRNA 1, primary spheres,P=6.5 × 10−3,n=5, secondary spheres,P=9.8 × 10−3,n=5; shRNA 2, primary spheres,P=8.0 × 10−3,n=6, secondary spheres,P=2.7 × 10−2,n=4; ANOVA). (c) Quantification of the percent of FOXG1-silenced BT025 and BT048 cells that incorporated BrdU compared with non-silenced cells (mean±s.e.m.; BT025: shRNA 1,P=2.2 × 10−3,n=7; shRNA 2,P=1.7 × 10−3,n=4; BT048, shRNA 1,P=1.1 × 10−3,n=5; shRNA 2,P=3.0 × 10−4,n=4; ANOVA). (d) Western blot analysis of PCNA and p21Cip1(p21) expression in non-silenced or FOXG1-silenced BT025 and BT048 cells. (e) Senescence-associated β-GALACTOSIDASE activity (pH, 6.0) in non-silenced or FOXG1-silenced BT025 cells. Top row, GFP fluorescence; bottom row, 5-bromo-4-chloro-3-indolyl-β-galactopyranoside (X-Gal) staining. Scale bar, 20 μm. (f) Quantification of the percent of FOXG1-silenced BT025 and BT048 cells positive for X-Gal staining compared with non-silenced cells (mean±s.e.m.; BT025: shRNA 1,P=6.1 × 10−3,n=5; shRNA 2,P=8.5 × 10−3,n=4; BT048: shRNA 1,P=2.7 × 10−2,n=4; shRNA 2,P=4.0 × 10−2,n=4; ANOVA). (g) Quantitative reverse transcription–PCR analysis of the indicated genes in non-silenced or FOXG1-silenced BT048 cells (mean±s.e.m.;p21Cip1,P=7.0 × 10−4;β-GALACTOSIDASE(β-Gal),P=1.3 × 10−2;GADD45A,P<1.0 × 10−4;n=3; ANOVA). (h) ChIP analysis ofp21Cip1,β-GALACTOSIDASEandGADD45Apromoter occupancy in BT025 and BT048 cells performed using rabbit anti-FOXG1 antibody or control rabbit immunoglobulin. Input genomic DNA (Input) was also subjected to PCR. DNA size standards are indicated in base pairs. One representative ChIP experiment is shown in each case (n≥3). Figure 3: FOXG1 silencing impairs proliferation in cultured BTICs. ( a ) Western blot analysis of FOXG1 in BTIC lines BT025 and BT048 after transduction with lentivirus expressing non-silencing shRNA or FOXG1 shRNA 1 and 2 reagents. β-ACTIN is shown as loading control. Molecular size markers are indicated in kDa. One representative western blot result is shown in each case ( n ≥3). ( b ) Quantification of the sphere-forming ability of non-silenced or FOXG1-silenced BT025 and BT048 cells passaged for two generations (mean±s.e.m. ; BT025: shRNA 1, primary spheres, P =2.0 × 10 −4 , n =10, secondary spheres, P =2.3 × 10 −3 , n =6; shRNA 2, primary spheres, P =9.1 × 10 −3 , n =3, secondary spheres, P =5.5 × 10 −3 , n =3; BT048: shRNA 1, primary spheres, P =6.5 × 10 −3 , n =5, secondary spheres, P =9.8 × 10 −3 , n =5; shRNA 2, primary spheres, P =8.0 × 10 −3 , n =6, secondary spheres, P =2.7 × 10 −2 , n =4; ANOVA). ( c ) Quantification of the percent of FOXG1-silenced BT025 and BT048 cells that incorporated BrdU compared with non-silenced cells (mean±s.e.m. ; BT025: shRNA 1, P =2.2 × 10 −3 , n =7; shRNA 2, P =1.7 × 10 −3 , n =4; BT048, shRNA 1, P =1.1 × 10 −3 , n =5; shRNA 2, P =3.0 × 10 −4 , n =4; ANOVA). ( d ) Western blot analysis of PCNA and p21 Cip1 (p21) expression in non-silenced or FOXG1-silenced BT025 and BT048 cells. ( e ) Senescence-associated β-GALACTOSIDASE activity (pH, 6.0) in non-silenced or FOXG1-silenced BT025 cells. Top row, GFP fluorescence; bottom row, 5-bromo-4-chloro-3-indolyl-β-galactopyranoside (X-Gal) staining. Scale bar, 20 μm. ( f ) Quantification of the percent of FOXG1-silenced BT025 and BT048 cells positive for X-Gal staining compared with non-silenced cells (mean±s.e.m. ; BT025: shRNA 1, P =6.1 × 10 −3 , n =5; shRNA 2, P =8.5 × 10 −3 , n =4; BT048: shRNA 1, P =2.7 × 10 −2 , n =4; shRNA 2, P =4.0 × 10 −2 , n =4; ANOVA). ( g ) Quantitative reverse transcription–PCR analysis of the indicated genes in non-silenced or FOXG1-silenced BT048 cells (mean±s.e.m. ; p21 Cip1 , P =7.0 × 10 −4 ; β-GALACTOSIDASE ( β-Gal ), P =1.3 × 10 −2 ; GADD45A , P <1.0 × 10 −4 ; n =3; ANOVA). ( h ) ChIP analysis of p21 Cip1 , β-GALACTOSIDASE and GADD45A promoter occupancy in BT025 and BT048 cells performed using rabbit anti-FOXG1 antibody or control rabbit immunoglobulin. Input genomic DNA (Input) was also subjected to PCR. DNA size standards are indicated in base pairs. One representative ChIP experiment is shown in each case ( n ≥3). Full size image We next examined the effect of FOXG1 silencing on the proliferation of BTICs cultured at higher cell-density, non-clonogenic, conditions [9] , [12] , [35] . FOXG1 silencing using two separate shRNA reagents caused a significant decrease in the number of S-phase BTICs that incorporated 5-bromodeoxyuridine (BrdU) compared with non-silenced cells ( Fig. 3c ). FOXG1 silencing also resulted in decreased expression of the proliferating-cell nuclear antigen (PCNA) marker and a converse upregulation of the cell cycle inhibitor CDKN1a/p21 Cip1 (p21 Cip1 hereafter; Fig. 3d ; for quantification, see Supplementary Fig. S4c ). In addition to increased p21 Cip1 levels, FOXG1 knockdown caused a significant increase in the frequency of BTICs positive for cytoplasmic β-GALACTOSIDASE activity ( Figs. 3e,f ). The change in p21 Cip1 protein expression was paralleled by a similar increase in transcript levels ( Fig. 3g ). Interestingly, mRNA levels of β-GALACTOSIDASE were also increased ( Fig. 3g ). Increases in p21 Cip1 level and β-GALACTOSIDASE activity were shown to be common hallmarks of cellular senescence [36] , [37] , [38] , suggesting that FOXG1 knockdown may promote cell cycle exit and replicative senescence in cultured BTICs. In agreement with this possibility, FOXG1 silencing also caused an upregulation of growth arrest and DNA damage-inducible 45A ( GADD45A ), a gene involved in cellular senescence together with p21 Cip1 (refs 38 , 39 ; Fig. 3g ). Chromatin immunoprecipitation (ChIP) experiments demonstrated further that endogenous FOXG1 localized to the promoters of p21 Cip1 , β-GALACTOSIDASE and GADD45A in BTICs ( Fig. 3h ), suggesting that FOXG1 may repress these genes in BTICs. The role of FOXG1 in the repression of p21 Cip1 expression is in agreement with previous studies in other cell types [28] , [40] . Together, these results suggest that FOXG1 promotes proliferation in cultured BTICs, at least in part, by preventing cell cycle exit and replicative senescence. FOXG1 silencing promotes astroglial gene expression in BTICs We next examined whether the decreased proliferative capacity of FOXG1-silenced BTICs was correlated with an increased propensity to activate neural differentiation programmes. This possibility was also suggested by the observation that the expression of endogenous FOXG1 was decreased alongside that of the NSPC markers SOX2, BMI1 and OLIG2 when BTICs were switched from self-renewing and non-differentiative culture conditions to conditions promoting in vitro differentiation [12] , [35] ( Fig. 4a ; for quantification, see Supplementary Fig. S5a ). Silencing of FOXG1 in BTICs maintained under non-differentiative conditions resulted in decreased levels of SOX2, BMI1 and OLIG2, showing that the knockdown of FOXG1 was sufficient to recapitulate the changes induced by a switch to differentiative culture conditions ( Fig. 4b ; for quantification, see Supplementary Fig. S5a ). ChIP experiments revealed that endogenous FOXG1 was localized to the promoter regions of both SOX2 and BMI1 , raising the possibility that FOXG1 is important for the activation/consolidation of the expression of these genes in BTICs ( Fig. 4c ). The latter finding is in agreement with the recent demonstration that FOXG1 can bind to the BMI1 promoter in medulloblastoma-derived tumour-initiating cells [41] . 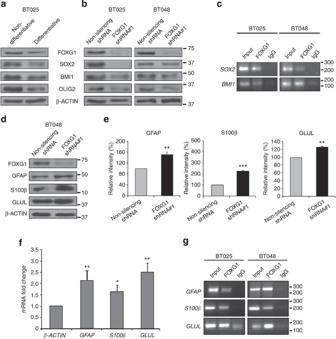Figure 4: FOXG1 silencing promotes expression of astroglial genes in BTICs. (a) Western blot analysis of the indicated proteins in BTIC line BT025 cultured under non-differentiative or differentiative conditions. β-ACTIN is shown as loading control. One representative western blotting result is shown in each case (n≥3). (b) Western blot analysis of the indicated proteins in non-silenced or FOXG1-silenced BT025 and BT048 cells (cultured under non-differentiative conditions). Molecular size markers are indicated in kDa. (c) ChIP analysis ofSOX2andBMI1promoter occupancy in BT025 and BT048 cells using rabbit anti-FOXG1 antibody or rabbit pre-immune immunoglobulin. Input genomic DNA (Input) was also subjected to PCR. DNA size standards are indicated in base pairs. One representative ChIP experiment is shown in each case (n≥3). (d) Western blot analysis of the expression of the indicated proteins in BT048 cells (cultured under non-differentiative conditions) after transduction with lentiviral vectors expressing non-silencing shRNA orFOXG1shRNA 1. GLUL, GLUTAMINE SYNTHETASE. (e) Quantification of western blotting data from separate experiments performed in BT048 cells, similar to the one shown ind. Data are represented as mean±s.e.m. (GFAP,P=8.0 × 10−3; S100β,P=2.4 × 10−5; GLUL,P=1.8 × 10−3;n=3;t-test). (f) Quantitative reverse transcription–PCR analysis of the indicated genes in BT048 cells after transduction with lentiviral vectors expressing non-silencing shRNA orFOXG1shRNA 1. Values are expressed as fold change ofFOXG1shRNA-transduced cells over non-silencing shRNA-transduced cells usingβ-ACTINas control (mean±s.e.m.;GFAP,P=6.7 × 10−3;S100β,P=1.7 × 10−2;GLUL,P=2.7 × 10−3;n=3; analysis of variance). (g) ChIP analysis ofGFAP,S100βandGLULpromoter occupancy in BT025 and BT048 cells performed using rabbit anti-FOXG1 antibody or control rabbit immunoglobulin, followed by PCR with primers specific for each of these genes. Input genomic DNA (Input) was subjected to PCR with the same primers. Figure 4: FOXG1 silencing promotes expression of astroglial genes in BTICs. ( a ) Western blot analysis of the indicated proteins in BTIC line BT025 cultured under non-differentiative or differentiative conditions. β-ACTIN is shown as loading control. One representative western blotting result is shown in each case ( n ≥3). ( b ) Western blot analysis of the indicated proteins in non-silenced or FOXG1-silenced BT025 and BT048 cells (cultured under non-differentiative conditions). Molecular size markers are indicated in kDa. ( c ) ChIP analysis of SOX2 and BMI1 promoter occupancy in BT025 and BT048 cells using rabbit anti-FOXG1 antibody or rabbit pre-immune immunoglobulin. Input genomic DNA (Input) was also subjected to PCR. DNA size standards are indicated in base pairs. One representative ChIP experiment is shown in each case ( n ≥3). ( d ) Western blot analysis of the expression of the indicated proteins in BT048 cells (cultured under non-differentiative conditions) after transduction with lentiviral vectors expressing non-silencing shRNA or FOXG1 shRNA 1. GLUL, GLUTAMINE SYNTHETASE. ( e ) Quantification of western blotting data from separate experiments performed in BT048 cells, similar to the one shown in d . Data are represented as mean±s.e.m. (GFAP, P =8.0 × 10 −3 ; S100β, P =2.4 × 10 −5 ; GLUL, P =1.8 × 10 −3 ; n =3; t -test). ( f ) Quantitative reverse transcription–PCR analysis of the indicated genes in BT048 cells after transduction with lentiviral vectors expressing non-silencing shRNA or FOXG1 shRNA 1. Values are expressed as fold change of FOXG1 shRNA-transduced cells over non-silencing shRNA-transduced cells using β-ACTIN as control (mean±s.e.m. ; GFAP , P =6.7 × 10 −3 ; S100β , P =1.7 × 10 −2 ; GLUL , P =2.7 × 10 −3 ; n =3; analysis of variance). ( g ) ChIP analysis of GFAP , S100β and GLUL promoter occupancy in BT025 and BT048 cells performed using rabbit anti-FOXG1 antibody or control rabbit immunoglobulin, followed by PCR with primers specific for each of these genes. Input genomic DNA (Input) was subjected to PCR with the same primers. Full size image Concomitant with a decreased expression of undifferentiated neural lineage markers, FOXG1 knockdown caused an increase in the levels of GFAP , S100β and GLUTAMINE SYNTHETASE , three genes usually found in combination in developing/developed astrocytes. These changes were observed at both mRNA and protein levels in two different BTIC lines ( Fig. 4d–f and Supplementary Fig. S5b,c ). We demonstrated further that endogenous FOXG1 was localized to the promoters of GFAP , S100β and GLUTAMINE SYNTHETASE in BTICs, consistent with a direct involvement of FOXG1 in the regulation of these genes in BTICs ( Fig. 4g ). We also observed that the level of the neuronal marker protein type III β-tubulin decreased in FOXG1-silenced BTICs, whereas no significant changes were detected in the expression of 2′,3′-cyclic-nucleotide 3′-phosphodiesterase and galactocerebroside, two proteins expressed in developing/developed oligodendrocytes ( Supplementary Fig. S5d,e ). Taken together, these results provide evidence, suggesting that FOXG1 participates in mechanisms that suppress the activation of selected astroglial differentiation programmes in cultured BTICs. FOXG1 silencing decreases BTIC-initiated tumour growth On the basis of the previous results, we examined whether FOXG1 silencing would impair the growth of brain tumours initiated by cultured BTICs following intracranial transplantation into host mice. BTIC line BT048 (ref. 12 ) expressing green fluorescent protein (GFP) together with either non-silencing or FOXG1 shRNA was stereotactically injected into the right striatum of recipient NOD-SCID (non-obese diabetic/severe combined immunodeficient) mice, followed by whole-mount analysis of GFP expression to visualize the implanted cells. Mice that had received FOXG1-silenced BT048 cells ( n =7 mice) consistently exhibited smaller GFP-positive tumours compared with mice injected with non-silenced BT048 cells ( n =8 mice) 10 weeks after implantation ( Fig. 5a,b ). Tumours initiated by BT048 cells were generally quite invasive and infiltrated the overlying cortex and migrated along the corpus callosum ( Fig. 5c ). Cell-counting studies in the latter region, chosen as an anatomically well-defined structure where implanted cells could be accurately counted, showed that the number of GFP-positive tumour cells was significantly smaller in mice that received FOXG1 -silenced BT048 cells compared with mice implanted with non-silenced cells ( Fig. 5c–e ). Importantly, analysis of survival rates showed that the smaller size of tumours initiated by FOXG1-silenced BT048 cells was correlated with a significant prolongation of survival of the transplanted mice compared with mice injected with non-silenced cells ( Fig. 5f ). To confirm these results, similar studies were performed using a separate BTIC line, BT025 (ref. 12 ). Mice that had received FOXG1-silenced BT025 cells also exhibited smaller GFP-expressing tumours and survived significantly longer compared with mice implanted with non-silenced BT025 cells ( Fig. 5g,h ). Primary cultures of neurosphere-forming cells derived from brain tumours explanted from mice injected with FOXG1-silenced BTICs exhibited a reduced sphere-forming ability compared with cells derived from tumours explanted from mice injected with non-silenced BTICs ( Fig. 5i ). This situation was correlated with increased levels of p21 Cip1 expression in the xenograft-derived FOXG1-silenced neurosphere-forming cells ( Fig. 5j ). Together, these results provide evidence that FOXG1 is important for the growth of BTIC-propagated brain tumours in vivo . 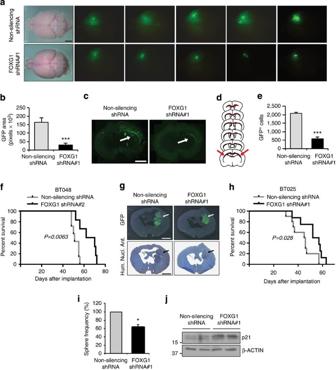Figure 5: FOXG1 silencing decreases BTIC-initiated brain tumour growth. (a–e) Comparison of brain tumour growth in NOD-SCID (non-obese diabetic/severe combined immunodeficient) mice euthanized 10 weeks after implantation of BTIC line BT048 transduced with lentivirus encoding GFP together with either non-silencing shRNA orFOXG1shRNA 1. (a) First column shows dorsal view of a pair of representative brains. All other columns show whole-mount GFP expression in five separate implanted brains. Scale bar, 2 mm. (b) Quantification of GFP expression across the dorsal brain of implanted mice as an area of green pixels using Adobe Photoshop (mean±s.e.m.;P=1.43 × 10−4;n=5;t-test). (c) GFP expression in coronal sections through the forebrain of implanted mice. Arrows point to location of tumour cells. Scale bar, 2 mm. (d) Representation of coronal sections through different levels of the forebrain used for cell-counting studies; arrows point to thecorpus callosum. (e) Graph depicting the number of GFP-expressing tumour cells in thecorpus callosumof the forebrain of implanted mice. Cell counts are based on six coronal sections through equivalent locations of separate brains (mean±s.e.m.;P=1.02 × 10−4;n=3 brains;t-test). (f) Kaplan–Meier survival curves of mice implanted with non-silenced or FOXG1-silenced (shRNA 2) BT048 cells (non-silencing shRNA,n=8 mice;FOXG1shRNA 2,n=7 mice). Statistical analysis (P-value) is shown (Mantel–Cox test). (g) Expression of GFP and human nuclear antigen in tumour cells in coronal sections through the forebrain of mice implanted with non-silenced or FOXG1-silenced (shRNA 1) BTIC line BT025. Arrows point to location of tumour cells. Scale bar, 2 mm. (h) Kaplan–Meier survival curves of mice implanted with non-silenced or FOXG1-silenced (shRNA 1) BT025 cells (non-silencing shRNA,n=10 mice;FOXG1shRNA 1,n=9 mice). Statistical analysis (P-value) is shown (Mantel–Cox test). (i) Quantification of the neurosphere-forming ability of primary cultures derived from brain cancers formed in host mice implanted with BT025 cells expressing non-silencing shRNA orFOXG1shRNA 1 (mean±s.e.m.;P=2.3 × 10−2;n=3;t-test). (j) Western blot analysis of p21Cip1expression in neurosphere-forming cells derived from brain cancers propagated in host mice by BT025 cells expressing non-silencing shRNA orFOXG1shRNA 1 (two examples are shown in each case). Molecular size markers are indicated in kDa. Figure 5: FOXG1 silencing decreases BTIC-initiated brain tumour growth. ( a – e ) Comparison of brain tumour growth in NOD-SCID (non-obese diabetic/severe combined immunodeficient) mice euthanized 10 weeks after implantation of BTIC line BT048 transduced with lentivirus encoding GFP together with either non-silencing shRNA or FOXG1 shRNA 1. ( a ) First column shows dorsal view of a pair of representative brains. All other columns show whole-mount GFP expression in five separate implanted brains. Scale bar, 2 mm. ( b ) Quantification of GFP expression across the dorsal brain of implanted mice as an area of green pixels using Adobe Photoshop (mean±s.e.m. ; P =1.43 × 10 −4 ; n =5; t -test). ( c ) GFP expression in coronal sections through the forebrain of implanted mice. Arrows point to location of tumour cells. Scale bar, 2 mm. ( d ) Representation of coronal sections through different levels of the forebrain used for cell-counting studies; arrows point to the corpus callosum . ( e ) Graph depicting the number of GFP-expressing tumour cells in the corpus callosum of the forebrain of implanted mice. Cell counts are based on six coronal sections through equivalent locations of separate brains (mean±s.e.m. ; P =1.02 × 10 −4 ; n =3 brains; t -test). ( f ) Kaplan–Meier survival curves of mice implanted with non-silenced or FOXG1-silenced (shRNA 2) BT048 cells (non-silencing shRNA, n =8 mice; FOXG1 shRNA 2, n =7 mice). Statistical analysis ( P -value) is shown (Mantel–Cox test). ( g ) Expression of GFP and human nuclear antigen in tumour cells in coronal sections through the forebrain of mice implanted with non-silenced or FOXG1-silenced (shRNA 1) BTIC line BT025. Arrows point to location of tumour cells. Scale bar, 2 mm. ( h ) Kaplan–Meier survival curves of mice implanted with non-silenced or FOXG1-silenced (shRNA 1) BT025 cells (non-silencing shRNA, n =10 mice; FOXG1 shRNA 1, n =9 mice). Statistical analysis ( P -value) is shown (Mantel–Cox test). ( i ) Quantification of the neurosphere-forming ability of primary cultures derived from brain cancers formed in host mice implanted with BT025 cells expressing non-silencing shRNA or FOXG1 shRNA 1 (mean±s.e.m. ; P =2.3 × 10 −2 ; n =3; t -test). ( j ) Western blot analysis of p21 Cip1 expression in neurosphere-forming cells derived from brain cancers propagated in host mice by BT025 cells expressing non-silencing shRNA or FOXG1 shRNA 1 (two examples are shown in each case). Molecular size markers are indicated in kDa. Full size image TLE functionally interacts with FOXG1 in cultured BTICs To characterize the molecular mechanisms underlying FOXG1 function in GBM and BTICs, we focused on the demonstrated interaction of FOXG1 with the transcriptional corepressor TLE in brain cells [23] , [24] , [25] . TLE expression, characterized by immunohistochemistry with previously validated anti-TLE (‘panTLE’) antibodies [42] , [43] , [44] , was broadly detected in human normal brain, grade II and grade III glioma and GBM specimens ( Fig. 6a ), consistent with the previous demonstration that TLE is expressed in many cell types, including neurons and glia [25] , [26] , [42] , [43] , [44] . Western blot analysis showed that TLE protein levels were higher in GBM compared with normal brain ( Supplementary Fig. S6a ). TLE-expressing cells also expressed GFAP, SOX2, NESTIN and BMI1 in GBM specimens, as well as in cultured BTICs; in the latter, we detected expression of TLE1 and TLE2 ( Supplementary Fig. S6b–d ). Importantly, virtually all TLE-positive cells coexpressed FOXG1 in GBM tissues (95.8±2.9%; mean±s.e.m., n =5) and cultured BTICs ( Fig. 6b ). Analysis of the GeneSapiens database showed that TLE1 mRNA levels were elevated in glioma compared with other tumours ( Fig. 6c ). This situation was correlated with a decrease in overall survival of GBM patients in the presence of increased TLE1 expression ( Fig. 6d ), similar to the situation associated with elevated FOXG1 . TLE2 was not detectably upregulated in glioma and no significant correlation between TLE2 levels and overall GBM patient survival was revealed by the REMBRANDT database ( Supplementary Fig. S6e,f ). 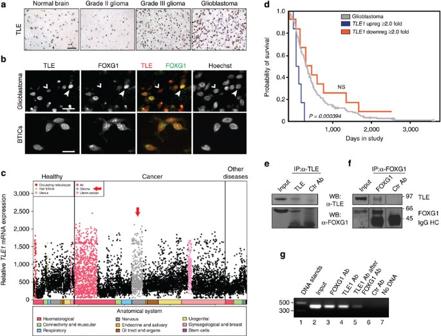Figure 6: TLE is expressed in GBM and BTICs. (a) Formalin-fixed, paraffin-embedded sections from the indicated specimens were subjected to immunohistochemistry with panTLE antibody, followed by counterstaining with haematoxylin (normal brain,n=13; grade II glioma,n=12; grade III glioma,n=16; GBM,n=16). A representative image is shown for each group. Scale bar, 50 μm. (b) Double-labelling immunofluorescence analysis of TLE and FOXG1 in GBM or cultured BT012 cells. Nuclei were counterstained with Hoechst. Closed arrowhead: example of cell with overlapping expression; open arrowhead: example of TLE-positive/FOXG1-negative cell. Scale bar, 20 μm. The same results were obtained in BTIC line BT048 (Supplementary Fig. S6d). (c) Body-wide expression ofTLE1across the GeneSapiens database, with each dot representing expression in a single sample. Anatomical sources of examined samples are indicated with coloured bars below the gene plot, with corresponding legends also shown. Anatomical samples with higher-than-averageTLE1expression or an outlier expression profile are shown coloured. Vertical red arrow points toTLE1expression in glioma. (d) Kaplan–Meier curves for GBM patients with tumours exhibiting either high (blue curve) or low (orange curve)TLE1mRNA levels compared with all GBM patients (grey curve). Data were obtained from the Rembrandt Database of the National Cancer Institute. Statistical analysis (P-value calculated using Mantel–Cox test) for high versus allTLE1levels is shown next to the corresponding curve. (e) Immunoprecipitation from BT048 cells using rabbit anti-TLE1 or control (Ctr) rabbit antibodies, followed by western blotting with anti-FOXG1 and anti-TLE antibodies. Input lysate (1/10) was also analysed. Molecular size markers are indicated in kDa. One representative result is shown (n≥3). (f) Immunoprecipitation using rabbit anti-FOXG1 or control rabbit antibodies, followed by western blotting with anti-TLE and anti-FOXG1 antibodies. Input lysate (1/10) was also analysed. IgG HC, immunoglobulin G heavy chain. (g) Either single (lanes 3 and 4) or sequential (lane 5) ChIP analysis ofp21Cip1promoter occupancy in BT048 cells using anti-FOXG1, anti-TLE1 or control antibodies. Controls also included omission of genomic DNA (No DNA). Input genomic DNA (Input) was also subjected to PCR. DNA standards (Stands) are shown and their size is indicated in base pairs. One representative ChIP experiment is presented (n≥3). Figure 6: TLE is expressed in GBM and BTICs. ( a ) Formalin-fixed, paraffin-embedded sections from the indicated specimens were subjected to immunohistochemistry with panTLE antibody, followed by counterstaining with haematoxylin (normal brain, n =13; grade II glioma, n =12; grade III glioma, n =16; GBM, n =16). A representative image is shown for each group. Scale bar, 50 μm. ( b ) Double-labelling immunofluorescence analysis of TLE and FOXG1 in GBM or cultured BT012 cells. Nuclei were counterstained with Hoechst. Closed arrowhead: example of cell with overlapping expression; open arrowhead: example of TLE-positive/FOXG1-negative cell. Scale bar, 20 μm. The same results were obtained in BTIC line BT048 ( Supplementary Fig. S6d ). ( c ) Body-wide expression of TLE1 across the GeneSapiens database, with each dot representing expression in a single sample. Anatomical sources of examined samples are indicated with coloured bars below the gene plot, with corresponding legends also shown. Anatomical samples with higher-than-average TLE1 expression or an outlier expression profile are shown coloured. Vertical red arrow points to TLE1 expression in glioma. ( d ) Kaplan–Meier curves for GBM patients with tumours exhibiting either high (blue curve) or low (orange curve) TLE1 mRNA levels compared with all GBM patients (grey curve). Data were obtained from the Rembrandt Database of the National Cancer Institute. Statistical analysis ( P -value calculated using Mantel–Cox test) for high versus all TLE1 levels is shown next to the corresponding curve. ( e ) Immunoprecipitation from BT048 cells using rabbit anti-TLE1 or control (Ctr) rabbit antibodies, followed by western blotting with anti-FOXG1 and anti-TLE antibodies. Input lysate (1/10) was also analysed. Molecular size markers are indicated in kDa. One representative result is shown ( n ≥3). ( f ) Immunoprecipitation using rabbit anti-FOXG1 or control rabbit antibodies, followed by western blotting with anti-TLE and anti-FOXG1 antibodies. Input lysate (1/10) was also analysed. IgG HC, immunoglobulin G heavy chain. ( g ) Either single (lanes 3 and 4) or sequential (lane 5) ChIP analysis of p21 Cip1 promoter occupancy in BT048 cells using anti-FOXG1, anti-TLE1 or control antibodies. Controls also included omission of genomic DNA (No DNA). Input genomic DNA (Input) was also subjected to PCR. DNA standards (Stands) are shown and their size is indicated in base pairs. One representative ChIP experiment is presented ( n ≥3). Full size image Immunoprecipitation of endogenous TLE from cultured BTICs resulted in the coprecipitation of endogenous FOXG1 and, conversely, TLE coprecipitated with endogenous FOXG1 when the latter was immunoprecipitated ( Fig. 6e,f ). In addition, sequential ChIP experiments in which protein:DNA complexes were precipitated using anti-FOXG1 antibody first, followed by anti-TLE1 antibody, demonstrated that both of these proteins were present on the same region of the p21 Cip1 promoter in BTICs ( Fig. 6g ). Together, these findings demonstrate that FOXG1 is coexpressed with the transcriptional corepressor TLE in GBM, and that these proteins form endogenous complexes in BTICs. TLE knockdown phenocopies FOXG1 silencing in BTICs To determine whether TLE was a functionally significant partner of FOXG1 in BTICs, we first tested whether knockdown of endogenous TLE in these cells would phenocopy at least some of the consequences of FOXG1 silencing. The sphere-forming ability of three separate lines of BTICs was significantly reduced as a result of TLE1 silencing using two separate shRNA reagents ( Fig. 7a,b and Supplementary Fig. S7a,b ). Moreover, TLE1 knockdown resulted in a significant upregulation of p21 Cip1 expression and a converse decrease in cell proliferation, as demonstrated by reduced PCNA expression and BrdU incorporation ( Fig. 7c,d and Supplementary Fig. S7c–f ). The same results were obtained when TLE2 was knocked down using two separate shRNA reagents ( Fig. 7a–d and Supplementary Fig. S7g–i ). We also observed that endogenous TLE1 and FOXG1 were localized to the same region of the promoters of β-GALACTOSIDASE and GADD45A ( Fig. 7e ), analogous to the situation detected with the p21 Cip1 promoter. Together, these findings provide evidence that, similar to FOXG1 TLE is involved in mechanisms important for the propagation of BTICs. 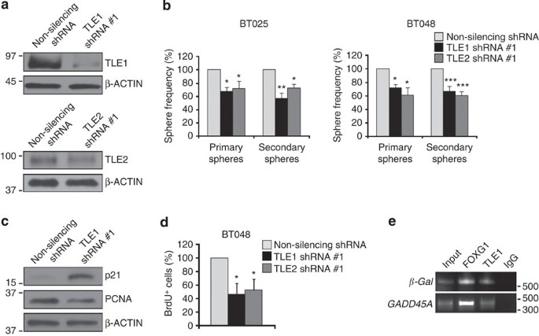Figure 7: TLE knockdown phenocopies the effects of FOXG1 silencing in BTICs. (a) Western blot analysis of TLE1 or TLE2 in BT048 cells after transduction with lentivirus expressing non-silencing shRNA,TLE1shRNA 1 orTLE2shRNA 1. β-ACTIN is shown as loading control. (b) Quantification of the sphere-forming ability of non-silenced, TLE1-silenced (shRNA 1), or TLE2-silenced (shRNA 1) BT025 and BT048 cells passaged for two generations (mean±s.e.m.; BT025:TLE1shRNA 1, primary spheres,P<1.1 × 10−2,n=4, secondary spheres,P=5.9 × 10−3,n=4;TLE2shRNA 1, primary spheres,P=1.8 × 10−2,n=5, secondary spheres,P=4.4 × 10−2,n=3; BT048:TLE1shRNA 1, primary spheres,P=4.7 × 10−2,n=4, secondary spheres,P=4.0 × 10−4,n=4;TLE2shRNA 1, primary spheres,P=1.8 × 10−2,n=3, secondary spheres,P=2.0 × 10−4,n=3; analysis of variance (ANOVA)). (c) Western blot analysis of p21Cip1(p21) and PCNA expression in non-silenced or TLE1-silenced (shRNA 1) BT048 cells. (d) Quantification of the percent of TLE1-silenced (shRNA 1) or TLE2-silenced (shRNA 1) BT048 cells that incorporated BrdU compared with non-silenced cells (mean±s.e.m.;TLE1shRNA 1,P=2.3 × 10−2;TLE2shRNA 1,P=3.9 × 10−2,n=4; ANOVA). (e) ChIP analysis ofβ-GALACTOSIDASE(β-Gal) andGADD45Apromoter occupancy in BT048 cells performed using rabbit anti-FOXG1, rabbit anti-TLE1 or control rabbit immunoglobulin. Input genomic DNA (Input) was also subjected to PCR. DNA size standards are indicated in base pairs. One representative ChIP experiment is shown in each case (n≥3). Figure 7: TLE knockdown phenocopies the effects of FOXG1 silencing in BTICs. ( a ) Western blot analysis of TLE1 or TLE2 in BT048 cells after transduction with lentivirus expressing non-silencing shRNA, TLE1 shRNA 1 or TLE2 shRNA 1. β-ACTIN is shown as loading control. ( b ) Quantification of the sphere-forming ability of non-silenced, TLE1-silenced (shRNA 1), or TLE2-silenced (shRNA 1) BT025 and BT048 cells passaged for two generations (mean±s.e.m. ; BT025: TLE1 shRNA 1, primary spheres, P <1.1 × 10 −2 , n =4, secondary spheres, P =5.9 × 10 −3 , n =4; TLE2 shRNA 1, primary spheres, P =1.8 × 10 −2 , n =5, secondary spheres, P =4.4 × 10 −2 , n =3; BT048: TLE1 shRNA 1, primary spheres, P =4.7 × 10 −2 , n =4, secondary spheres, P =4.0 × 10 −4 , n =4; TLE2 shRNA 1, primary spheres, P =1.8 × 10 −2 , n =3, secondary spheres, P =2.0 × 10 −4 , n =3; analysis of variance (ANOVA)). ( c ) Western blot analysis of p21 Cip1 (p21) and PCNA expression in non-silenced or TLE1-silenced (shRNA 1) BT048 cells. ( d ) Quantification of the percent of TLE1-silenced (shRNA 1) or TLE2-silenced (shRNA 1) BT048 cells that incorporated BrdU compared with non-silenced cells (mean±s.e.m. ; TLE1 shRNA 1, P =2.3 × 10 −2 ; TLE2 shRNA 1, P =3.9 × 10 −2 , n =4; ANOVA). ( e ) ChIP analysis of β-GALACTOSIDASE ( β-Gal ) and GADD45A promoter occupancy in BT048 cells performed using rabbit anti-FOXG1, rabbit anti-TLE1 or control rabbit immunoglobulin. Input genomic DNA (Input) was also subjected to PCR. DNA size standards are indicated in base pairs. One representative ChIP experiment is shown in each case ( n ≥3). Full size image FOXG1:TLE antagonist GRG6 impairs proliferation in BTICs To further investigate whether FOXG1 could form complexes with TLE important for the regulation of BTIC behaviour, we took advantage of the previous demonstration that the TLE-related protein GRG6 binds with high affinity to FOXG1 but not other known TLE transcription partners tested to date [24] , [45] . Contrary to TLE, however, GRG6 does not have transcription repression activity. As a result, GRG6 can act as a dominant-negative inhibitor of the transcription repression functions of FOXG1:TLE complexes when expressed at high-enough levels to compete with TLE for FOXG1 binding [24] ( Fig. 8a ). We showed that FOXG1 and GRG6 formed complexes when coexpressed in GBM cell lines ( Supplementary Fig. S8a ). Using a validated anti-GRG6 antibody ( Supplementary Fig. S8b,c ), we observed that both the number of GRG6-expressing cells ( Fig. 8b,c ) and the GRG6 expression level ( Fig. 8d ) were considerably higher in normal brain compared with GBM, in contrast to the situation observed with FOXG1, and also contrary to the robust expression of TLE in GBM. 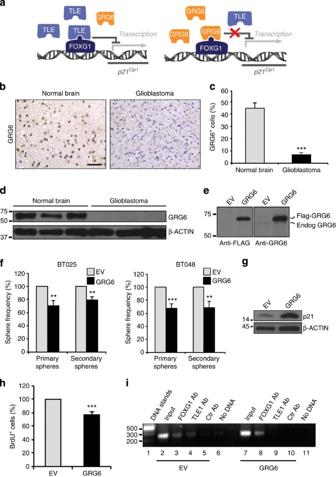Figure 8: GRG6 overexpression phenocopies the effects of FOXG1 and TLE silencing in BTICs. (a) Model of antagonistic contributions of TLE and GRG6 to FOXG1 transcription repression activity. FOXG1 mediates transcriptional repression of target genes (for example,p21Cip1) when in a complex with TLE. The transcription repression activity of FOXG1:TLE can be antagonized by GRG6, which can compete with TLE for FOXG1 binding but does not have transcriptional corepressor activity. (b) Formalin-fixed, paraffin-embedded sections from normal brain (n=13) or GBM (n=15) tissues were subjected to immunohistochemistry with anti-GRG6 antibody, followed by counterstaining with haematoxylin. A representative image is shown for each group. Scale bar, 50 μm. (c) Quantification of the percent of GRG6-positive nuclei in normal brain or GBM specimens (mean±s.e.m.; GBM,P=6.8 × 10−8;n=13; normal brain,n=10;t-test). (d) Western blot analysis of endogenous GRG6 expression in normal brain and GBM specimens, as indicated. β-ACTIN is shown as loading control. Molecular size markers are indicated in kDa. (e) Western blot analysis of BT048 cells using anti-FLAG epitope or anti-GRG6 antibodies following transduction with FLAG-GRG6-expressing lentivirus or empty vector (EV) control lentivirus. Exogenous GRG6 exhibits retarded mobility compared with endogenous (Endog) GRG6 due to the FLAG epitope. One representative result is shown (n≥3). (f) Quantification of the sphere-forming ability of BT025 and BT048 cells passaged for two generations after transduction with empty vector or GRG6 lentivirus (mean±s.e.m.; BT025, primary spheres,P=1.1 × 10−3, secondary spheres,P=1.5 × 10−3; BT048, primary spheres,P=1.7 × 10−4, secondary spheres,P=6.2 × 10−3;n≥5;t-test). (g) Western blot analysis of p21Cip1(p21) expression in BT048 cells after transduction with EV or GRG6 lentivirus. (h) Quantification of the percent of BT048 cells that incorporated BrdU after transduction with GRG6 lentivirus compared with EV lentivirus (mean±s.e.m.;P=3.1 × 10−4;n=7;t-test). (i) ChIP analysis ofp21Cip1promoter occupancy in BT048 cells transduced with either empty vector (lanes 2–5) or GRG6 (lanes 7–10) lentivirus. Experiments were performed using rabbit anti-FOXG1 (lanes 3 and 8), rabbit anti-TLE1 (lanes 4 and 9) or control (Ctrl) rabbit (lanes 5 and 10) antibodies, followed by PCR amplification with primers specific for thep21promoter. Input genomic DNA (Input; lanes 2 and 7) was subjected to PCR with the same primers. DNA standards (Stands, lane 1) are shown and their size indicated in base pairs. One representative ChIP experiment is shown (n≥3). Figure 8: GRG6 overexpression phenocopies the effects of FOXG1 and TLE silencing in BTICs. ( a ) Model of antagonistic contributions of TLE and GRG6 to FOXG1 transcription repression activity. FOXG1 mediates transcriptional repression of target genes (for example, p21 Cip1 ) when in a complex with TLE. The transcription repression activity of FOXG1:TLE can be antagonized by GRG6, which can compete with TLE for FOXG1 binding but does not have transcriptional corepressor activity. ( b ) Formalin-fixed, paraffin-embedded sections from normal brain ( n =13) or GBM ( n =15) tissues were subjected to immunohistochemistry with anti-GRG6 antibody, followed by counterstaining with haematoxylin. A representative image is shown for each group. Scale bar, 50 μm. ( c ) Quantification of the percent of GRG6-positive nuclei in normal brain or GBM specimens (mean±s.e.m. ; GBM, P =6.8 × 10 −8 ; n =13; normal brain, n =10; t -test). ( d ) Western blot analysis of endogenous GRG6 expression in normal brain and GBM specimens, as indicated. β-ACTIN is shown as loading control. Molecular size markers are indicated in kDa. ( e ) Western blot analysis of BT048 cells using anti-FLAG epitope or anti-GRG6 antibodies following transduction with FLAG-GRG6-expressing lentivirus or empty vector (EV) control lentivirus. Exogenous GRG6 exhibits retarded mobility compared with endogenous (Endog) GRG6 due to the FLAG epitope. One representative result is shown ( n ≥3). ( f ) Quantification of the sphere-forming ability of BT025 and BT048 cells passaged for two generations after transduction with empty vector or GRG6 lentivirus (mean±s.e.m. ; BT025, primary spheres, P =1.1 × 10 −3 , secondary spheres, P =1.5 × 10 −3 ; BT048, primary spheres, P =1.7 × 10 −4 , secondary spheres, P =6.2 × 10 −3 ; n ≥5; t -test). ( g ) Western blot analysis of p21 Cip1 (p21) expression in BT048 cells after transduction with EV or GRG6 lentivirus. ( h ) Quantification of the percent of BT048 cells that incorporated BrdU after transduction with GRG6 lentivirus compared with EV lentivirus (mean±s.e.m. ; P =3.1 × 10 −4 ; n =7; t -test). ( i ) ChIP analysis of p21 Cip1 promoter occupancy in BT048 cells transduced with either empty vector (lanes 2–5) or GRG6 (lanes 7–10) lentivirus. Experiments were performed using rabbit anti-FOXG1 (lanes 3 and 8), rabbit anti-TLE1 (lanes 4 and 9) or control (Ctrl) rabbit (lanes 5 and 10) antibodies, followed by PCR amplification with primers specific for the p21 promoter. Input genomic DNA (Input; lanes 2 and 7) was subjected to PCR with the same primers. DNA standards (Stands, lane 1) are shown and their size indicated in base pairs. One representative ChIP experiment is shown ( n ≥3). Full size image On the basis of these observations, exogenous GRG6 was significantly overexpressed in cultured BTICs via lentiviral-mediated delivery ( Fig. 8e ), to determine whether this manipulation would have effects analogous to the knockdown of FOXG1 or TLE. Exogenous GRG6 expression resulted in decreased sphere-forming ability in three separate BTIC lines ( Fig. 8f and Supplementary Fig. S8d ). Forced expression of exogenous GRG6 in these cells also caused increased expression of p21 Cip1 , decreased BrdU incorporation ( Fig. 8g,h ) and reduced PCNA levels ( Supplementary Fig. S8e ). These effects were correlated with a downregulation of markers of the undifferentiated neural state, such as BMI1, and an upregulation of GFAP expression in BTICs ( Supplementary Fig. S8e ). ChIP experiments showed further that although GRG6 overexpression did not affect the binding of FOXG1 to the p21 Cip1 promoter in these cells, it resulted in a detectable decrease in the recruitment of TLE to the same promoter region, consistent with the ability of GRG6 to compete with TLE for FOXG1 binding ( Fig. 8i ). Experiments aimed at determining whether GRG6 was recruited to the p21 Cip1 promoter in place of TLE proved technically unfeasible due to the lack of ChIP-quality anti-GRG6 antibodies. Taken together, these findings show that GRG6 overexpression has the same effects on BTIC behaviour as the silencing of FOXG1 or TLE, suggesting that GRG6 has the potential to act as an antagonist of FOXG1:TLE transcription repression complexes in BTICs. GRG6 overexpression decreases BTIC-initiated tumour growth On the basis of the previous results, we compared the growth of brain tumours initiated by control or GRG6-overexpressing BTICs after intracranial transplantation into host mice. Tumours initiated by GRG6-overexpressing BT025 cells were smaller compared with tumours derived from BT025 cells transduced with empty vector lentivirus when examined at equivalent endpoints ( Fig. 9a ). Consistent with these observations, mice harbouring brain tumours originated from GRG6-overexpressing BT025 cells survived significantly longer compared with control mice ( Fig. 9b ). The same result was obtained when GRG6 was overexpressed before intracranial transplantation in a second BTIC line, BT012 (ref. 12 ; Fig. 9c ). Tumour xenografts initiated by a third GRG6-overexpressing BTIC line, BT048, were also smaller than tumours derived from control BT048 cells ( Supplementary Fig. S9a ). Moreover, primary cultures of neurosphere-forming cells derived from resected GRG6-overspressing tumours propagated by both BT025 and BT048 cells exhibited persistently elevated expression of exogenous GRG6, decreased sphere-forming ability in vitro and increased p21 Cip1 levels when compared with cells derived from tumours initiated by control BTICs ( Fig. 9d,e and Supplementary Fig. S9b,c ). Altogether, these results show that increased levels of GRG6 reduce the growth of BTIC-propagated brain tumours in vivo , similar to the effect of FOXG1 silencing. 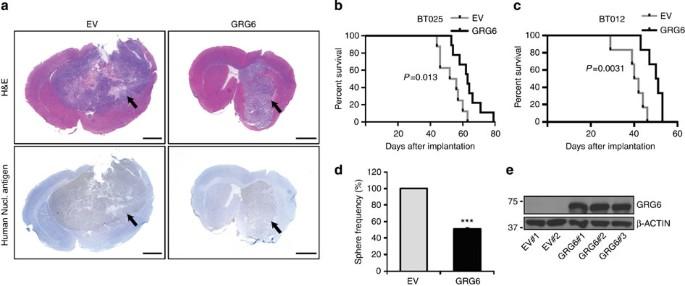Figure 9: GRG6 overexpression decreases BTIC-initiated brain tumour growth. (a) Representative images of coronal sections through the forebrain of NOD-SCID (non-obese diabetic/severe combined immunodeficient) mice that reached clinical endpoints at equivalent days after stereotactical implantation of BTIC line BT025 transduced with empty vector (EV) (n=8) or GRG6-encoding (n=10) lentivirus. In this example, brains were collected either 52 (EV) or 53 (GRG6) days after implantation. Top row depicts staining with haematoxylin and eosin (H&E). Bottom row depicts immunohistochemistry with anti-human-specific nuclear antigen antibody. Arrows point to location of brain tumours. Scale bar, 2 mm. (b,c) Kaplan–Meier survival curves of mice implanted with either BT025 (b) or BT012 (c) cells transduced with EV or GRG6-encoding lentivirus. In each case, two groups of implanted mice were maintained until they were found to have succumbed to tumour burden or developed neurological symptoms that required euthanasia (BT025: EV,n=8; GRG6,n=10; BT012: EV,n=6; GRG6,n=6). Statistical analysis (P-value) is shown (Mantel–Cox test). (d) Quantification of the neurosphere-forming ability of primary cultures derived from three separate brain tumours formed in host mice implanted with BT025 cells transduced with EV- or GRG6-encoding lentivirus. Data are shown as mean±s.e.m. (P=2.5 × 10−5;n=3;t-test). (e) Western blot analysis of exogenous GRG6 expression in neurosphere-forming cells derived from brain tumours that grew in mice implanted with BT025 cells transduced with empty vector- or GRG6 lentivirus. Molecular size markers are indicated in kDa. Figure 9: GRG6 overexpression decreases BTIC-initiated brain tumour growth. ( a ) Representative images of coronal sections through the forebrain of NOD-SCID (non-obese diabetic/severe combined immunodeficient) mice that reached clinical endpoints at equivalent days after stereotactical implantation of BTIC line BT025 transduced with empty vector (EV) ( n =8) or GRG6-encoding ( n =10) lentivirus. In this example, brains were collected either 52 (EV) or 53 (GRG6) days after implantation. Top row depicts staining with haematoxylin and eosin (H&E). Bottom row depicts immunohistochemistry with anti-human-specific nuclear antigen antibody. Arrows point to location of brain tumours. Scale bar, 2 mm. ( b , c ) Kaplan–Meier survival curves of mice implanted with either BT025 ( b ) or BT012 ( c ) cells transduced with EV or GRG6-encoding lentivirus. In each case, two groups of implanted mice were maintained until they were found to have succumbed to tumour burden or developed neurological symptoms that required euthanasia (BT025: EV, n =8; GRG6, n =10; BT012: EV, n =6; GRG6, n =6). Statistical analysis ( P -value) is shown (Mantel–Cox test). ( d ) Quantification of the neurosphere-forming ability of primary cultures derived from three separate brain tumours formed in host mice implanted with BT025 cells transduced with EV- or GRG6-encoding lentivirus. Data are shown as mean±s.e.m. ( P =2.5 × 10 −5 ; n =3; t -test). ( e ) Western blot analysis of exogenous GRG6 expression in neurosphere-forming cells derived from brain tumours that grew in mice implanted with BT025 cells transduced with empty vector- or GRG6 lentivirus. Molecular size markers are indicated in kDa. Full size image Understanding the molecular mechanisms that govern the behaviour of BTICs is considered a key step towards the design of new therapeutic strategies that may improve current treatment options for GBM [5] , [9] , [10] , [14] , [46] . However, the mechanisms underlying BTIC pathobiology remain only partly defined. In this study, we have provided previously unavailable evidence for an important role of the transcription factors FOXG1 and TLE in the regulation of BTIC-initiated brain tumour growth, implicating these proteins in GBM tumourigenesis. The present results have shown that FOXG1 is robustly expressed in GBM, where many FOXG1-expressing cells display molecular features of poorly differentiated astroglial cells. This situation is different from non-cancerous adult brain, where FOXG1-expressing cells in the parenchyma outside the subventricular zone correspond to postmitotic neurons. We detected FOXG1 expression in all GBM cases examined, suggesting that FOXG1 is not associated with a particular adult GBM subtype. This finding is consistent with the recent observation that FOXG1 is expressed in four GBM subgroups displaying gene expression profiles typical of proneural, mesenchymal, classical and mixed subtypes based on DNA methylation data and their correlations with mutational status, DNA copy-number aberrations and gene expression signatures [29] . Our studies have shown further that FOXG1 is expressed in both actively mitotic and more quiescent cells in GBM. At least a fraction of the latter may correspond to NSPC-like cells, because we detected overlap of FOXG1 expression with the expression of a number of NSPC markers in GBM specimens. Moreover, FOXG1 is expressed in cultured GBM-derived BTICs rigorously selected on the basis of their in vitro stem-like properties and in vivo tumourigenic potential, even when transplanted at very low numbers [12] . Silencing of FOXG1 in cultured BTICs results in decreased sphere-forming ability and BrdU incorporation, with a concomitant upregulation of genes associated with cell cycle exit and replicative senescence, such as p21 Cip1 and GADD45A , as well as β-GALACTOSIDASE , whose activity is known to increase in senescent cells [37] , [38] , [39] , [40] . We have shown further that endogenous FOXG1 binds to the promoters of the latter three genes in BTICs. Together, these observations suggest that FOXG1 is important for sustained BTIC proliferation, at least in part, by repressing the expression of genes that promote cessation of proliferation and replicative senescence. FOXG1 knockdown in BTICs also leads to decreased expression of markers typical of the undifferentiated NSPC state, including OLIG2 , SOX2 and BMI1 . Endogenous FOXG1 is recruited to the promoters of both SOX2 and BMI1 in BTICs. The latter finding is consistent with the recent observation that FOXG1 binds to the BMI1 promoter in medulloblastoma stem-like cells and that knockdown of FOXG1 causes decreased BMI1 transcription in these cells [41] . The decreased expression of NSPC markers caused by FOXG1 silencing in BTICs is associated with a converse upregulation of three genes commonly present in developing/developed astrocytes, namely GFAP , S100β and glutamine synthetase . Endogenous FOXG1 binds to the promoters of these genes, directly implicating FOXG1 in the transcriptional regulation of GFAP , S100β and glutamine synthetase in BTICs. Taken together with the demonstrated involvement of mouse Foxg1 in NSPC maintenance and inhibition of astrocyte differentiation [21] , these findings suggest that FOXG1 is involved in the maintenance of the undifferentiated state and the suppression of astrocyte cell lineage differentiation in BTICs. In agreement with these observations, in vivo orthotopic transplantation studies have demonstrated that brain tumours initiated by FOXG1-silenced BTICs are smaller than tumours initiated by non-silenced BTICs, resulting in prolonged host survival. This finding provides evidence that FOXG1 has an important role in BTIC-propagated brain tumour growth. This possibility is consistent with the demonstration that increased Foxg1 expression in the developing mouse brain causes forebrain hypercellularity resulting from increased progenitor cell expansion and delayed differentiation [22] . The involvement of FOXG1 in the tumourigenic potential of BTICs is also in agreement with the previous association of FOXG1 with various cancers. The chicken orthologue of FOXG1 was originally characterized as the avian sarcoma virus oncogene, qin [47] . Moreover, FOXG1 is overexpressed in human hepatoblastoma and medulloblastoma [41] , [48] , [49] , as well as in ovarian cancer [40] . In some of these tumours, FOXG1 is hypothesized to sustain cell proliferation, at least in part, by repressing transcription of cell cycle inhibitory genes like p21 Cip1 (refs 28 , 40 , 50 ), similar to the situation observed in BTICs. In transfected epithelial cell lines, the ability of FOXG1 to antagonize p21 Cip1 gene activation was proposed to result from the recruitment of FOXG1 to the p21 Cip1 promoter in association with FOXO3:SMAD2/3 transcription complexes. It was proposed that these latter complexes activate the p21 Cip1 promoter in response to transforming growth factor-β (TGF-β) signalling and that FOXG1 suppresses their transactivation activity, thereby acting as an antagonist of the cytostatic effects of TGF-β. [28] However, it seems unlikely that FOXG1 promotes BTIC maintenance and tumourigenic potential by antagonizing TGF-β signalling, because previous work has shown that similar to the roles of FOXG1 described in this study, TGF-β increases proliferation and prevents differentiation in BTICs [13] . The converse possibility that FOXG1 and TGF-β signalling might cooperate to maintain BTICs remains to be determined. We have shown further that FOXG1 forms complexes in BTICs with the transcriptional corepressor TLE, a key partner of FOXG1 during rodent and amphibian forebrain development [23] , [24] , [25] . FOXG1 and TLE localize together to the same region of the p21 Cip1 promoter in BTICs, and silencing of FOXG1 or TLE results in a similar upregulation of p21 Cip1 expression. Similarly, both FOXG1 and TLE are bound to common regions within the GADD45A and β-GALACTOSIDASE promoters. Moreover, the negative effect of FOXG1 silencing on the proliferative ability of BTICs can be phenocopied by TLE1 or TLE2 knockdown. These findings suggest that at least some of the functions of FOXG1 in BTICs involve the formation of transcription repression complexes with TLE proteins. This possibility is further supported by the results of our studies of GRG6, a transcription repression-incompetent antagonist of the functions of FOXG1:TLE complexes [24] . We have shown that GRG6 expression is low in GBM and robust in normal brain, in contrast to the high expression of both FOXG1 and TLE in GBM. More importantly, experimental protocols resulting in a forced overexpression of GRG6 in BTICs cause a significant decrease in the proliferation and tumourigenic potential of these cells, equivalent to the effects of FOXG1 knockdown. It should be emphasized that it is unlikely that the effects of GRG6 overexpression in BTICs were caused by a general inhibition of TLE functions. GRG6 shares with TLE a carboxyl-terminal WD-40 repeat domain that mediates interactions with several transcription factors, including FOXG1 (ref. 26 ). GRG6 binds to FOXG1 through its WD-40 repeat domain with a similar affinity to that of TLE. However, GRG6 fails to bind to, or interacts only poorly with, several other TLE-binding partners tested to date [24] , [45] . In addition, GRG6 does not contain the amino-terminal Gln-rich domain that is used by TLE as a second protein–protein interaction surface [26] . As a result, GRG6 is not a general antagonist of all TLE functions; rather, its restricted protein–protein interaction capacity makes GRG6 a more selective dominant inhibitor of transcription complexes involving FOXG1 and, possibly, other FOXG1-related proteins. In summary, the present studies define the expression of FOXG1 and TLE in human GBM and BTICs. Moreover, they provide important information on the roles of these proteins in BTIC proliferation, differentiation and tumour-forming ability, as well as the molecular mechanisms underlying their functions in these cells. Furthermore, they suggest that at least certain components of the transcriptional programmes regulated by FOXG1 and TLE in BTICs are important for the tumour-forming ability of these cells. Some of the FOXG1 and TLE target genes may be specific to BTICs and not shared with normal NSPCs, thus providing possible targets for efforts to impair the tumorigenic potential of BTICs with the aim of providing novel advances in the fight against GBM. Patient data sets and Kaplan–Meier survival plot Relative FOXG1 mRNA expression data in different human cancers were obtained from the public version of the GeneSapiens Database ( http://www.genesapiens.org ). Survival data for glioma patients were publicly available in de-identified form on the Rembrandt database website ( https://caintegrator.nci.nih.gov/rembrandt/ ) using data available on 4 September 2012. Kaplan–Meier survival curves were generated for GBM patients ( n =181) using microarray data from the Affymetrix U133 Plus 2.0 GeneChip and associated survival data. The ‘highest geometric mean intensity’ of FOXG1 was used as the reporter for relative FOXG1 expression within the database. FOXG1 up- or downregulation was defined as at least a twofold difference from the mean expression level within a given data set. No institutional review board approval was needed, because the use of these data was not classified as human subject research. BTIC culture BTICs were isolated and cultured from GBM surgical specimens (after informed consent was obtained) as previously described [12] . Briefly, extensively rinsed tumour specimens were finely minced and placed in DMEM/Ham’s F12 (1:1) (Invitrogen) containing 5 mM HEPES buffer, 0.6% glucose, 3 mM sodium bicarbonate, 2 mM glutamine, 25 μg ml −1 insulin, 100 μg ml −1 transferrin, 20 nM progesterone, 10 μM putrescine and 30 nM selenite (Sigma-Aldrich). A series of mechanical dissociations was used to obtain a single-cell suspension, followed by filtration through a 40-μm filter. Cells were resuspended in serum-free culture medium (NeuroCult medium, StemCell Technologies) and plated at a density of 20,000 viable cells per ml. Brain tumour-derived neurospheres were evident as early as 1 week after plating. Spheres were grown for at least 3 weeks or until they reached a size ( ~ 100–200 μm) adequate for plating and passaging. The phenotype of these cells was confirmed by scoring for prolonged in vitro propagation under clonogenic conditions, NSPC marker expression and in vivo tumour initiation ability, according to previously published protocols [12] and as described in more detail in sections below. The same protocols were used to re-derive new primary BTIC cultures from orthotopic tumour xenografts propagated by BTICs BT025 and BT048 implanted into host mice. Immunohistochemistry and immunofluorescence Frozen and formalin-fixed, paraffin-embedded sections of de-identified adult human normal brain ( n =13), inflamed brain ( n =4) and glioma ( n =12 for grade II, n =16 for grade III and n =30 for GBM) specimens were obtained from the Department of Pathology of Treviso Hospital (University of Padova, Treviso, Italy), the Department of Pathology of McGill University (Montreal, QC, Canada) and the Canadian Brain Tumour Tissue Bank (London Health Sciences Centre, London, ON, Canada). Normal brain and glioma specimens were derived, respectively, from temporal lobectomy for epilepsy surgery or tumour resection of primary glioma. Inflamed brain specimens were obtained during abscess or encephalitis surgeries. For paraffin-embedded tissues, sections were subjected to the removal of paraffin, rehydration and citrate-based (pH, 6.0) antigen retrieval, blocking and incubation with anti-FOXG1 (1:1,000), anti-TLE (1:10) or anti-GRG6 (1:1,000) antibodies. A horseradish peroxidase-based Vectastain ABC kit using 3,3′-diaminobenzidine substrate (Vector Laboratories Inc.) was used for the detection of primary antibodies. Nuclei were counterstained with haematoxylin. A similar procedure was used with frozen human surgical specimens or mouse tumour xenografts, except that neither removal of paraffin nor antigen retrieval was required. Immunofluorescence staining of tissue sections or adherent BTICs was performed as described previously [51] , [52] . Briefly, samples were rinsed twice in PBS and then pre-incubated for 1 h in blocking solution, which consisted of 5% normal donkey serum (Jackson ImmunoResearch Laboratories), 0.1% Triton-X-100 and 0.5 mg ml −1 BSA (Sigma-Aldrich) in PBS. Sections were then incubated for 2 h at room temperature or 16 h at 4 °C in blocking solution containing the following primary antibodies: rabbit anti-FOXG1 (1:1,000; Abcam, number Ab18259) [53] , mouse anti-BMI1 (1:100, Millipore, number 05-637), goat anti-SOX2 (1:100; R&D Syst., number AF2018), mouse anti-OLIG2 (1:300; Millipore, number MABN50), mouse anti-human NESTIN (1:1,000; Millipore, number MAB5326), mouse anti-GFAP (1:1,000; Sigma-Aldrich, number G3893), mouse anti-Ki67 (1:800; BD Pharmingen, number 556003), mouse anti-CD44 (1:100; BD Pharmingen, number 550392), mouse anti-NeuN (1:100; Millipore, number MAB377), rat anti-TLE (‘panTLE’) (1:10) [42] , [43] , [44] or mouse anti-GRG6 (1:1,000; Abnova, number H00079816-M01). The fluorescent-conjugated secondary antibodies used included the Alexa Fluor 488 and 555 series (1:1,000; Molecular Probes). Counterstaining was performed with Hoechst 33258 (Sigma-Aldrich). Images were acquired using either a Digital Video Camera mounted on a Zeiss Axioskop 2 microscope or a Retiga EXi Camera (Qimaging) on a Zeiss Axioscope Imager.M1 microscope. Images were digitally assigned to the appropriate red, green or blue channels using Northern Eclipse image acquisition software (Empix Imaging Inc.). Lentiviral trasduction of BTICs For knockdown studies, bicistronic lentiviral particles expressing enhanced GFP with either a control, non-silencing shRNA reagent (catalogue number RHS-4348) or shRNA sequences targeting human FOXG1 (sense sequence 1: 5′-ATGGGACCAGACTGTAAGTGAA-3′, Clone ID V3LHS_407592; sense sequence 2: 5′-CCAGCTCCGTGTTGACTCAGAA-3′, Clone ID V3LHS_353952), TLE1 (sense sequence 1: 5′-AGCAGTCTCCACTTGGCAATAA-3′, Clone ID V2LHS_18400; sense sequence 2: 5′-AATTATATCCGTTCCTGTA-3′, Clone ID V2LHS_18937), or TLE2 (sense sequence 1: 5′-TGCATTGATATTTCCGATT-3′, Clone ID V3LHS_360390; sense sequence 2: 5′-CAGCACTCCTGCCTCCAAA-3′, Clone ID V2LHS_171324) were obtained from Open Biosystems. For overexpression studies, lentiviral particles expressing a FLAG epitope-tagged form of human GRG6 (catalogue number LP-Z6833-Lv102), or empty vector control lentivirus (catalogue number LP-NEG-LV105-0200), were acquired from GeneCopoeia Inc. All of these lentiviral vectors conferred puromycin resistance to the transduced cells. Low-passage number BTICs were transduced at a multiplicity of infection of five and were analysed either 72 h post infection or after 1 week of selection in puromycin (1 μg ml −1 ). Transduction efficiency was determined by quantitating the amount of GFP-positive cells by FACS analysis (on average between 95 and 99% of cells expressed GFP). Sphere formation and BrdU incorporation assays The sphere-forming ability of BTIC lines BT012, BT025 and BT048 cultured at clonogenic density (100 cells per ml) was determined by quantification of the number of primary and secondary spheres (diameter ≥100 μm) as described [12] . Briefly, primary spheres were mechanically dissociated into single-cell suspensions. After cell counting, cells were replated under the original growth condition. Cultures were observed weekly for secondary sphere formation. BrdU incorporation experiments were performed by incubating BTICs cultured at high cell density (100,000 cells per ml) under previously described conditions [12] , [35] , in the presence of BrdU (3 μg ml −1 ) for 5 h at 37 °C, followed by immunofluorescence analysis using anti-BrdU antibody (1:200; Abcam, number Ab6326). BTIC differentiation BTICs were seeded on poly( L -ornithine)-coated culture dishes and induced to differentiate by addition of 1% fetal bovine serum to the culture medium for 7 days [12] . After this time, cells were harvested and lysed in 50 mM Tris–HCl, pH 7.8, 150 mM NaCl, 1 mM EDTA, 1% sodium deoxycholate, 0.1% SDS and 1% Triton-X-100 (supplemented with protease inhibitors). Lysates were then subjected to western blot analysis. Western blotting The following antibodies were used: rabbit anti-FOXG1 (1:1,000), goat anti-SOX2 (1:400), mouse anti-BMI1 (1:1,000), rabbit anti-OLIG2 (1:500; Abcam, number Ab81093), mouse anti-PCNA (1:1,000; Santa Cruz Biotech., number sc-56), mouse anti-p21 Cip1 (1:500; Dako, number M7202), mouse anti-GFAP (1:2,000, Sigma-Aldrich, number G3893), mouse anti-glutamine synthetase (1:2,000; Millipore, number MAB302), mouse anti-S100β (1:500; Sigma-Aldrich, number S2532), mouse anti-type III β-tubulin (1:2,000; Promega, number G712A), mouse anti-2′,3′-cyclic-nucleotide 3′-phosphodiesterase (1:2,000; Millipore, number MAB326R), mouse anti-galactocerebroside (1:500; Millipore, number MAB342), rabbit anti-TLE1 and anti-TLE2 (refs 44 , 54 , 55 , 56 ; 1:1,000), mouse anti-GRG6 (1:1,000) and mouse anti-β-ACTIN (1:10,000; Abcam, number Ab6276). Full-length images of western blots are shown in Supplementary Fig. S10 and S11 . Senescence analysis Senescence-associated β-galactosidase assays were performed using the Senescence β-galactosidase Staining Kit as per the manufacturer’s instructions (Cell Signaling, number 9860). BTIC implantation into immunocompromised mice Low-passage number BTICs were transduced with lentivirus expressing either non-silencing shRNA or FOXG1 shRNA 1 or 2 in one set of experiments or with empty vector- or FLAG-GRG6-expressing lentivirus in another experimental set. After 1 week of selection in the presence of puromycin (1 μg ml −1 ), cells were tested for successful FOXG1 silencing or GRG6 overexpression by western blotting. Cells were then mechanically dissociated to single-cell suspensions and subjected to cell counting using trypan blue to quantify viable cells, followed by resuspension of 1 × 10 5 or 5 × 10 5 cells (depending on experiments, as detailed below) in 3 μl of PBS. Intracranial implantation into the corpus striatum of the right hemisphere of 6- to 8-week-old CB-17 NOD-SCID male mice (Charles-River Laboratory) was performed exactly as described [12] . Coordinates for stereotactic implantation were as follows: anteroposterior −1.0, mediolateral 2.0 and dorsoventral 3.0. Survival experiments (5 × 10 5 cells were implanted) were terminated when animals succumbed to tumour burden or required euthanasia due to manifestation of neurological symptoms or significant loss of body weight. In experiments where tumour growth was compared (1 × 10 5 cells were implanted), mice were euthanized 10 weeks after implantation. Dissected brains were rinsed in PBS, followed by fixation, cryopreservation and embedding in Tissue-Tek OCT compound (Sakura Finetek) as described [51] , [52] . Frozen tissues were cryostat-sectioned (14 μm), mounted onto SuperFrost glass slides (Fisher) and stored at −20 °C until use. Whole-mount analysis of GFP expression in implanted brains was performed using a fluorescent Zeiss Discovery V.20 dissecting microscope. The human origin of the tumour xenografts was confirmed by immunohistochemistry with anti-human nuclear antigen antibody (1:200; Millipore). Animal procedures were conducted in accordance with the guidelines of the Canadian Council for Animal Care and were approved by the Animal Care Committee of the Montreal Neurological Institute of McGill University. Cell-counting studies The numbers of GFP-positive cells in the corpus callosum of brains from mice implanted with BTICs were counted every sixth coronal sections of 14 μm each (every 84 μm) derived from three different brains for each condition (at least 18 sections for each condition were analysed). Photo images were taken at × 20 magnification and full coronal photomontages, including the corpus callosum , were made using Microsoft ICE software. GFP-positive cells in the corpus callosum were counted using ImageJ software (US National Institutes of Health). Counts were performed over a volume of ~0.187208, mm 3 (across 6 sections). Chromatin immunoprecipitation ChIP experiments were performed using the Magna ChIP G kit (Millipore) following the manufacturer’s instructions. Chromatin of BTIC line BT048 was cross-linked with formaldehyde, sonicated to yield 300–500 bp fragments and subjected to immunoprecipitation using specific antibodies at a concentration of ~5 μg ml −1 . Protein:DNA complexes were harvested using protein-G magnetic beads and a magnetic separator, rinsed extensively and incubated at 62 °C in the presence of ‘ChIP Elution Buffer’ (Millipore) containing 0.1 mg ml −1 proteinase K to reverse the cross-linking and recover the DNA. Immunoprecipitated DNA was purified using spin columns supplied with the Magna ChIP G kit and then subjected to PCR. Sequential ChIP experiments were performed essentially as described [57] . Briefly, the protein:DNA products obtained using anti-FOXG1 antibody were recovered, extensively rinsed, eluted from the beads and then subjected again to ChIP using anti-TLE1 antibody or control antibodies. Washes, elution and crosslink reversal steps following the second immunoprecipitation were performed as in the case of non-sequential ChIP experiments. Immunoprecipitation reactions were performed with ChIP-grade rabbit anti-FOXG1 antibody (Abcam, number 18259), previously described anti-TLE1 antibody [44] , or pre-immune rabbit immunoglobulin (Cell Signaling, number 2729S). In the experiments depicted in Figs 6g and 8i , rabbit anti-inducible nitric oxide synthetase (Millipore, number AB1552) antibody was used as irrelevant, control, antibody. The complete list of oligonucleotide primers used in ChIP experiments is shown in Supplementary Table S1 . All PCR-amplified regions contained one or more consensus FOX-binding sites (A/TTGTTTA/T). Full-length images of DNA gels are shown in Supplementary Fig. S10 and S11 . Quantitative PCR Total RNA was isolated from BTICs using TRIzol reagent (Invitrogen, number 15596-026) and reverse transcribed using Bio-Rad iScript Reverse Transcription Supermix for quantitative reverse transcription–PCR (number 170-8840). Quantitative PCR was performed using the Bio-Rad CFX96 Touch Real-Time PCR Detection System using SsoFast EvaGreen Supermix (number 172-5201). Values were expressed as fold change of FOXG1 shRNA-transduced cells over non-silencing shRNA-transduced cells using β-ACTIN as a control, using the comparative CT method of analysis (means of three replicate experiments). The sequences of the oligonucleotides used in quantitative PCR experiments are listed in Supplementary Table S1 . Coimmunoprecipitation Immunoprecipitation of endogenous FOXG1 or TLE1 from lysates obtained from BTIC line BT048 was performed as described [44] , [45] using rabbit anti-FOXG1 antibody (Abcam, number Ab18259), rabbit anti-TLE1 antibody [44] , or control pre-immune rabbit immunoglobulin (Cell Signaling, number 2729S) at a concentration of 5–10 μg ml −1 . Immunoprecipitates, together with one out of ten of each input lysate, were analysed by western blotting using anti-FOXG1 and anti-TLE antibodies. Cell culture Malignant glioma cell lines U87MG and U251MG (obtained from the American Tissue Culture Collection) were cultured as monolayers in DMEM medium supplemented with 2 mM L -glutamine (Invitrogen) and 10% fetal bovine serum (Invitrogen). U251MG cells were transduced with lentiviral vectors expressing non-silencing shRNA or FOXG1 shRNA 1. U87MG cells were transfected using Lipofectamine 2000 (Invitrogen) with either control non-silencing small interfering RNA (siRNA; Dharmacon, number D-001810-10-05) or FOXG1 siRNA (Dharmacon, number L-019124-00). For coimmunoprecipitation studies, U87MG cells were transfected with plasmids pCMV2-FLAG-GRG6 and pCMV2-HA-FOXG1 (ref. 45 ), or their corresponding empty vectors as controls, followed by immunoprecipitation using anti-FLAG epitope antibody. Immunoprecipitates, together with 20% of each input lysate, were analysed by western blotting using anti-FLAG and anti-HA antibodies. HEK293 cells were transfected with non-silencing siRNA or GRG6 siRNA (Dharmacon, number LQ-014437-02). Statistical analysis Statistical comparisons were made using either analysis of variance followed by Dunnett’s post-hoc test or unpaired Student’s t -test, as indicated in the figure legends. Values were expressed as mean±s.e.m. Statistical tests were performed with Microsoft Excel and Prism v6.0 software. Survival curves were analysed using the Kaplan–Meier method with groups compared by respective median survival; log-rank P -value was measured using the Mantel–Cox test. Significance level was set at P <0.05. How to cite this article: Verginelli, F. et al. Transcription factors FOXG1 and Groucho/TLE promote glioblastoma growth. Nat. Commun. 4:2956 doi: 10.1038/ncomms3956 (2013).